Spectrally selective chiral silicon metasurfaces based on infrared Fano resonances Metamaterials and metasurfaces represent a remarkably versatile platform for light manipulation, biological and chemical sensing, and nonlinear optics. Many of these applications rely on the resonant nature of metamaterials, which is the basis for extreme spectrally selective concentration of optical energy in the near field. In addition, metamaterial-based optical devices lend themselves to considerable miniaturization because of their subwavelength features. This additional advantage sets metamaterials apart from their predecessors, photonic crystals, which achieve spectral selectivity through their long-range periodicity. Unfortunately, spectral selectivity of the overwhelming majority of metamaterials that are made of metals is severely limited by high plasmonic losses. Here we propose and demonstrate Fano-resonant all-dielectric metasurfaces supporting optical resonances with quality factors Q >100 that are based on CMOS-compatible materials: silicon and its oxide. We also demonstrate that these infrared metasurfaces exhibit extreme planar chirality, opening exciting possibilities for efficient ultrathin circular polarizers and narrow-band thermal emitters of circularly polarized radiation. Metasurfaces [1] , [2] are the two-dimensional single-layer counterparts of the fully three-dimensional metamaterials [3] , [4] . As their fabrication is considerably simpler in comparison with volumetric metamaterials, metasurfaces were the first to find practical applications at optical frequencies ranging from light manipulation [5] , [6] , [7] , [8] , [9] , [10] and sensing of minute analyte quantities [10] , [11] , [12] to nonlinear optics [13] , [14] , spectrally selective thermal emission [15] and even low-threshold lasing [16] . Many of these applications require photonic structures characterized by their highly spectrally selective response (corresponding to high-quality factor Q ), miniaturized format (preferably on the scale of no more than several wavelengths) and the convenience and high efficiency of far-field light coupling. The coupling efficiency issue, while seemingly mundane, is particularly important for mid-infrared applications because of the lack of ultrasensitive optical detectors in that frequency range. Simultaneously satisfying these requirements presents considerable challenge for most photonic structures. For example, the isolated high- Q microcavities reviewed in ref. 17 and suggested for biochemical sensing applications [18] , [19] suffer from poor far-field coupling [20] , [21] . Planar photonic crystals are also known to possess extremely spectrally selective optical responses (for example, reflection and transmission amplitudes or phases) [22] , [23] , [24] , [25] that have been exploited for various sensing [24] , [26] , [27] and filtering [22] applications. The very high-quality factors Q >1,000 (ref. 28 ) of such photonic resonances are often caused by the so-called guided resonance modes (GRMs) [22] , [23] , [29] . The spectrally narrow linewidth of these modes originates from the suppression of their radiative losses through the long-range destructive interference between multiple unit cells of a photonic crystal and, therefore, is extremely sensitive to the light’s incidence angle [22] , [24] , [25] , [28] , [30] , [31] . Such angular sensitivity prevents miniaturization of photonic crystal devices [22] , [26] , [32] and imposes severe restrictions on the angular divergence of the incident light beams. While highly collimated laser beams have been used for interrogating high-Q photonic crystal structures in the visible and telecommunication spectral ranges [25] , [26] , [31] , [33] , the angular divergence of incoherent beams used for mid-infrared spectroscopy is typically prohibitively high for utilizing GRMs supported by photonic crystals. Note that high angular sensitivity is also typical for the frequency-selective surfaces [34] that can be thought of as microwave predecessors [1] of metasurfaces. Metasurfaces avoid these limitations by employing a conceptually different design approach: its unit cell and its neighbouring interactions are engineered to reduce the combined radiative and non-radiative (that is, Ohmic) losses of the sharp resonances. Here the radiative losses are reduced by engineering the detailed geometry of the metasurface unit cells, while the non-radiative losses are reduced by judiciously selecting the unit cell material. One promising approach to decreasing radiative losses while maintaining finite coupling to free-space radiation is to utilize the phenomenon of Fano interference [35] originally introduced in atomic physics to describe asymmetrically shaped ionization spectral lines of atoms. More recently, the concept of Fano resonances was introduced to the field of photonics and metamaterials [23] , [28] , [36] , [37] , [38] , [39] in which a photonic structure possesses two resonances generally classified as ‘bright’ (that is, spectrally broad and strongly coupled to incident light) and ‘dark’ (spectrally sharp, with negligible radiative loss). The weak near-field coupling between the bright and dark resonances leads to coupling of the incident light to the dark resonance that maintains its low radiative loss, thereby remaining high- Q . Unfortunately, even for the most judicious engineering of the radiative loss, the total Q is limited [16] , [40] , [42] by the non-radiative loss of the underlying material. A notable exception is the special class of diffraction-coupled plasmonic arrays [25] , [43] , [44] , [45] , which rely on the geometric resonance that arises when the wavelength of light is commensurate with the array’s periodicity [44] . Such plasmonic arrays can possess a very high Q -factor, but suffer from the same limitations as GRM-based photonic crystals, affecting a number of important applications that involve ultrasmall (several wavelengths in size) samples. A typical example of such application is an infrared absorption sensor capable of resolving proteins’ secondary structure, which would require mid-infrared metamaterial resonances with Q ~\n100 to distinguish between their alpha-helical and beta-sheet conformations [46] that fall inside the Amide I (1,500 cm −1 < ω <1,700 cm −1 ) range. An equally important practical consideration is that the noble metals used for making high-Q plasmonic metasurfaces cannot be processed at CMOS-compatible fabrication facilities, thus limiting their scalability and standardization. One approach to reduce non-radiative losses without utilizing diffractive effects is to substitute metallic metamaterials by dielectric ones. Although the electromagnetic properties of dielectric resonators have been studied for decades [47] , [48] , [49] , all-dielectric infrared metamaterials have only recently been demonstrated [7] , [50] , [51] , [52] , [53] , and other non-metallic materials are being considered [54] . Despite this body of work, experimentally demonstrating sharp metamaterial resonances ( Q ~\n100) has proven to be challenging, thus greatly impeding further progress in applying metamaterials to practical problems such as biochemical sensing. Here we present an experimental realization of silicon-based infrared metasurfaces supporting Fano resonances with record-high quality factors Q >100. In addition, we experimentally demonstrate that high (>50%) linear-to-circular polarization conversion efficiency can be accomplished by making these silicon-based metasurfaces planar (2D) chiral [55] by design. Our supporting numerical simulations indicate that such metasurfaces can exhibit an extraordinary degree of planar chirality, thus opening exciting possibilities for developing narrow-band thermal emitters of circularly polarized radiation. Si-based metasurfaces are fabricated from standard commercially available silicon-in-insulator (SOI) wafers using standard CMOS-compatible semiconductor fabrication techniques, making them even more appealing for practical applications. Design of Si-based planar chiral metasurfaces The conceptual schematic of the metasurface used here and an SEM image of a typical sample are shown in Fig. 1 . The unit cell’s geometry is based on the earlier developed plasmonic metasurfaces that were utilized for plasmon-induced transparency [56] , protein monolayer sensing [12] and infrared spectroscopy of single-layer graphene (SLG) [57] . Each unit cell comprises one straight and one bent Si nanorods, where the bend is responsible for breaking the two mirror inversion symmetries of the unit cell and coupling the bright (electric dipole) and dark (electric quadrupole/magnetic dipole) resonances as schematically shown in Fig. 1c , where the surface charge density at the air/Si interface is plotted for the eigenmodes of the metasurfaces with and without a symmetry-breaking bend. 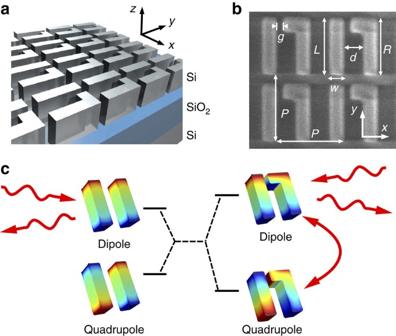Figure 1: Fano-resonant silicon metasurfaces. (a) A schematic of the silicon-based chiral metasurface supporting high-QFano resonances. (b) The SEM image of the fabricated sample and geometry definitions. Physical dimensions:P=2.4 μm,w=500 nm,d=700 nm,g=200 nm,R=2 μm and 1.6 μm<L<2 μm for the three samples that differ inL. (c) A schematic illustrating the Fano interference between electric dipolar (top left) and quadrupolar (bottom left) modes because of the symmetry-breaking small horizontal stub. The plotted colour-coded surface charge distributionsat the Si/air interfaces are calculated from eigenvalue simulations of the fields supported by the metasurface. The modes approximately retain their spatial symmetry after hybridization. Figure 1: Fano-resonant silicon metasurfaces. ( a ) A schematic of the silicon-based chiral metasurface supporting high- Q Fano resonances. ( b ) The SEM image of the fabricated sample and geometry definitions. Physical dimensions: P =2.4 μm, w =500 nm, d =700 nm, g =200 nm, R =2 μm and 1.6 μm< L <2 μm for the three samples that differ in L . ( c ) A schematic illustrating the Fano interference between electric dipolar (top left) and quadrupolar (bottom left) modes because of the symmetry-breaking small horizontal stub. The plotted colour-coded surface charge distributions at the Si/air interfaces are calculated from eigenvalue simulations of the fields supported by the metasurface. The modes approximately retain their spatial symmetry after hybridization. Full size image As collective interactions of each unit cell with its neighbours are important for imparting the metasurface with its optical properties, the eigenmodes of an infinite metasurface were calculated using finite element methods with the COMSOL software. More details on the interaction between neighbouring unit cells can be found in Supplementary Note 1 . Note [40] that the diffractive effects are unimportant in Fano-resonant metasurfaces, and the spectral position of the dark resonance is determined primarily by the unit cell’s geometry (its physical dimensions R , L , g , d and w shown in Fig. 1 ) and not by the period P separating them. Hybridization of the two resonances is responsible for the very sharp Fano features in transmission and reflection spectra as the dark resonance acquires a small electric dipole moment and strongly couples to the incident electromagnetic wave. The dark quadrupole resonance is not the only high-Q eigenmode supported by the metasurface. In fact, several strongly localized dark multipole resonances shown in Fig. 2 are supported. All resonances are computed for a metasurface with the period P =2.4 μm and nanorods’ cross-section of 0.5 μm × 1.2 μm in the x – z plane, with remaining dimensions given in the caption. On the basis of their spatial symmetry, the resonant modes are designated as TM ijk , with i , j , k =0 or 1 corresponding to the E y ( x, y, z ) being, respectively, even or odd under the x, y, z inversions. All dark modes are coupled in the near-field to the bright TM 000 mode, marked as ‘dipole’ in Fig. 1c . However, because the coupling of the higher-order dark modes to the TM 000 mode is even weaker than that of the lowest order TM 100 mode (marked in Fig. 1c as ‘quadrupole’), we expect, and experimentally confirm below, that these modes manifest in even sharper Fano resonances. Note that these modes are designated as dark because of their near-vanishing electric and magnetic dipole moments in the x – y plane and, consequently, weak coupling to the normally incident light. The degree of coupling is controlled by the design: a shorter symmetry-breaking bend of a nanorod would result in weaker coupling and higher quality factor Q. In contrast, the Q -factor of the bright modes possessing the in-plane electric/magnetic dipole moments cannot be arbitrarily increased because of the finite out-of-plane scattering that cannot be suppressed [53] , [58] . 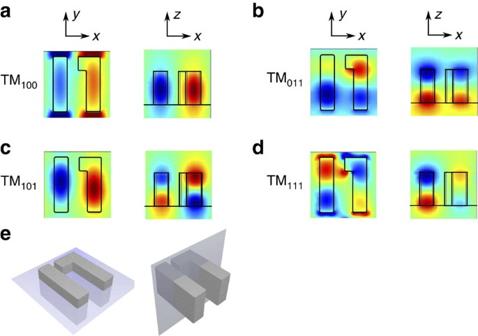Figure 2: Dark resonances supported by the silicon-based metasurface. (a–d) Colour maps ofEyin thex–yplane (left) andx–zplane (right). (e) Illustration of the cutting planes. Thex–yplane is atz=800 nm above the base of the silicon metasurface. Thex–zplane passes through the middle of the unit cell. The corresponding resonant wavelength areλ100=4.72 μm,λ011=4.21 μm,λ101=4.12 μm andλ111=4.07 μm, respectively. Physical dimensions of the metasurface: same as inFig. 1, withL=2 μm. Figure 2: Dark resonances supported by the silicon-based metasurface. ( a – d ) Colour maps of E y in the x – y plane (left) and x – z plane (right). ( e ) Illustration of the cutting planes. The x – y plane is at z =800 nm above the base of the silicon metasurface. The x – z plane passes through the middle of the unit cell. The corresponding resonant wavelength are λ 100 =4.72 μm, λ 011 =4.21 μm, λ 101 =4.12 μm and λ 111 =4.07 μm, respectively. Physical dimensions of the metasurface: same as in Fig. 1 , with L =2 μm. Full size image Experimental measurements of high- Q Fano resonances The experimental and numerical results presented in Fig. 3 , where the cross-polarized transmission spectra T ij ( λ ) were acquired using polarized infrared spectroscopy (see Methods for more details), are plotted as a function of the wavelength λ . The polarizations of the incident/transmitted light ( i , j = x or y ) are set by the polarizer/analyser, respectively, as shown in Fig. 4a . Spectral tunability of three representative metasurfaces was accomplished by varying the length 1.6 μm< L <2 μm of the left (straight) nanorod. The T yy ( λ ) spectra provide clear evidence of the Fano interference consistent with Fig. 1c : a broad dip at the frequency of the bright TM 000 mode at λ 000 ≈4.35 μm is superimposed on a set of narrow features corresponding to the dark modes shown in Fig. 2 . Similar Fano features are observed in the x -polarized transmission T xx ( λ ), where the broadband background reflectivity originates from the Fabry–Perot substrate resonances. 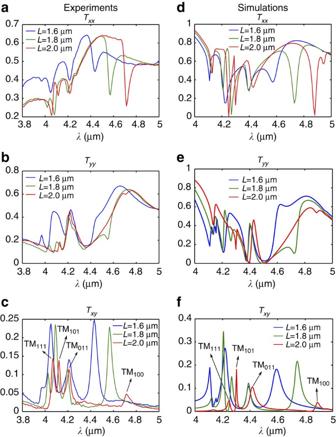Figure 3: Polarization-resolved transmission spectra of the silicon metasurfaces. Measured (a–c) and calculated (d–f) transmission spectra of the silicon metamaterials withL=1.6 μm (blue), 1.8 μm (green) and 2.0 μm (red). The spectra ofTxxare shown ina,d,Tyyare inb,eandTxyare inc,f. The four dark resonances are labelled inc,dfor theL=2 μm sample. Figure 3: Polarization-resolved transmission spectra of the silicon metasurfaces. Measured ( a – c ) and calculated ( d – f ) transmission spectra of the silicon metamaterials with L =1.6 μm (blue), 1.8 μm (green) and 2.0 μm (red). The spectra of T xx are shown in a , d , T yy are in b , e and T xy are in c , f . The four dark resonances are labelled in c , d for the L =2 μm sample. 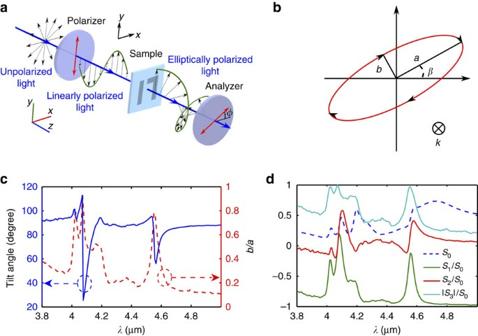Figure 4: Polarization state manipulation using Fano-resonant 2D chiral metasurfaces. (a) A schematic for the rotating analyser Stokes polarimetry. The incident beam is polarized in theydirection. (b) Definition of the polarization ellipse parameters. (c) The measured tilt angleβand the inverse of the ellipticityb/aof the polarization ellipse. (d) The measured Stokes parameters for theL=1.8 μm sample.S1,S2and |S3| are normalized with respect toS0. Unit cell dimensions: as inFig. 1andL=1.8 μm. Full size image Figure 4: Polarization state manipulation using Fano-resonant 2D chiral metasurfaces. ( a ) A schematic for the rotating analyser Stokes polarimetry. The incident beam is polarized in the y direction. ( b ) Definition of the polarization ellipse parameters. ( c ) The measured tilt angle β and the inverse of the ellipticity b/a of the polarization ellipse. ( d ) The measured Stokes parameters for the L =1.8 μm sample. S 1 , S 2 and | S 3 | are normalized with respect to S 0 . Unit cell dimensions: as in Fig. 1 and L =1.8 μm. Full size image The most remarkable spectral features are observed in the cross-polarized transmission T xy ( λ ). The baseline T xy ( λ ), small for all non-resonant wavelengths ( λ >5 μm), is dramatically peaked at Fano resonances, as shown in Fig. 3c,f , because of the coupling of the dark modes to both x and y polarizations of the incident light. The estimated quality factors Q = λ /Δ λ (where Δ λ is full-width half-maximum (FWHM) of each peak) of the Fano resonances, calculated by fitting the experimental cross-polarized spectra with Lorentzian curves, are listed in Table 1 for the three metasurfaces. Slightly more accurate values of the Q- factors can be obtained from the cross-polarized spectra [26] , [33] by fitting T xy ( λ ) to the standard Fano expression [35] as detailed in the Methods section. Table 1 Comparison of dark modes supported by the silicon metasurfaces. Full size table To our knowledge, these are the narrowest optical resonances observed in collective mid-IR metasurfaces that do not rely on diffractive effects that become important when the wavelength of light becomes commensurate with the periodicity of the array [44] . Unlike extremely angle-sensitive diffractive structures [22] , [24] , [25] , [28] , [44] , Fano-resonant metasurfaces are ideally matched to far-field radiation with moderate angular divergence Δ θ focused by low numerical aperture (NA) optics (Δ θ ≈7°and NA≈0.13 here). Such experimentally observed angular tolerance translates into minimum acceptable metasurface size W m ~\n λ /(2Δ θ ), which can be considerably smaller than W d ~\n Qλ /2 (ref. 22 ) (where λ is the wavelength of the infrared light) required for high- Q diffracting structures, such as those based on GRMs. Although achieving high- Q resonances depends on collective interactions [40] between neighbouring cells of the large area (300 μm × 300 μm) metasurfaces used in our experiments, our simulations confirm (see Supplementary Note 1 for details) that samples as small as 25 μm × 12.5 μm (or 6 λ × 3 λ ) can be utilized without any noticeable deterioration of the spectral sharpness. That is because only several neighbouring unit cells (two to three on each side horizontally, one on each side vertically according to Supplementary Note 1 ) effectively interact with each given unit cell. This short-range collective interaction contrasts with long-range coherence required for achieving narrow spectral width in photonic structures that rely on diffractive effects [44] , [45] . The unique capability to combine these small area high- Q metasurfaces with thermal infrared radiation sources is absolutely crucial for the future sensing applications described below. Experimental demonstration of linear-to-circular polarization conversion The first application of the planar (2D) chiral metasurfaces [55] described in this Article, suggested by the high cross-polarized transmission T xy , is efficient linear-to-circular polarization (LP-to-CP) conversion. The conversion efficiency and the degree of circular polarization (DCP) was experimentally investigated using the standard rotating analyser Stokes polarimetry setup [59] illustrated in Fig. 4a to characterize the transmitted polarization state of the y -polarized incident light, and to extract its Stokes parameters S 0 =| E x | 2 +| E y | 2 , S 1 =| E x | 2 −| E y | 2 , , and . A nonzero S 3 corresponds to elliptically polarized light, and S 3 =± S 0 corresponds to right/left CP light. Alternatively, the principal dimensions of the transmitted light’s polarization ellipse, its tilt angle β and the ratio a / b between its long and short axes defined in Fig. 4b , can be expressed in terms of the Stokes parameters (see the Methods section). The measured Stokes parameters and polarization ellipse dimensions for the metasurface with L =1.8 μm are plotted in Fig. 4c,d and are in good agreement with numerical simulations (see Supplementary Fig. 1 for comparisons and the data for the remaining metasurfaces). Note that, away from the Fano resonances, the polarization of the transmitted light is essentially unchanged from its original linear y -polarization, as expressed by S 1 / S 0 ≈−1 in Fig. 4d , and β ≈90°, b / a ≈0.1 in Fig. 4c for λ >4.7 μm. However, at the Fano resonances the polarization becomes essentially circular, as evidenced by | S 3 |/ S 0 ≈1 and b/a ≈0.8 at λ 100 ≈4.55 μm, with conversion efficiency S 0 ≈50%. Even a higher DCP ( b / a >0.9) is observed for the TM 101 mode at λ 101 ≈4.1 μm, thus demonstrating that these metasurfaces can be used for efficient narrow-band LP-to-CP conversion. Applications of chiral infrared metasurfaces The 2D chiral high-Q silicon metasurfaces described in this paper make them an attractive platform for a variety of applications that require spectral selectivity, small pixel size, relatively weak angular sensitivity and strong field enhancement. The simplicity and widespread availability of silicon fabrication techniques used in the semiconductor industry only add to the attractiveness of Si-based metasurfaces for practical applications. Recent advances [60] in transferring the otherwise stiff and brittle silicon structures on flexible substrates is another potentially important contributing factor to future adoption of Si-based metasurfaces by applications that require conformable or stretchable platforms. Below we outline two potential applications that are enabled by the metasurfaces described in this communication: one is the thermal emission of circularly polarized infrared radiation enabled by the extreme chirality of Si-based metasurfaces, and the other is sensing and bio-sensing enabled by the strong optical field concentration and spectral selectivity of these Fano-resonant metasurfaces. The 2D chiral nature of the metasurfaces discussed above lends itself to another unique application as a source of spectrally selective CP thermal infrared radiation [61] , which is uniquely distinct from the non-CP thermal radiation emitted by natural environments. Even though it is generally assumed that broadband CP emitters are desirable, high spectral selectivity is required for applications such as infrared identifiers (IRIDs) that rely on unique spectral and polarization signatures of infrared tags. Below we briefly outline the conceptual differences between 2D chiral metasurfaces [55] and other metamaterials used for LP-to-CP conversion, such as the recently demonstrated single-layer plasmonic quarter-wave plates [62] or chiral volumetric metamaterials [8] , [9] . The action of a quarter-wave plate is based on the phenomenon of birefringence, owing to which the two orthogonal polarizations of light acquire different phase shifts φ x,y in transmission. The incident LP light can be converted into an right-handed circularly polarized (RCP) or left-handed circularly polarized (LCP) polarization state in transmission if the phase difference Δ φ = φ x − φ y =± π /2. By changing the initial direction of the incoming linear polarization, either RCP or LCP state can be achieved. While quarter-wave plates based on birefringent metasurfaces can be used for efficient LP-to-CP polarization conversion, they cannot be used as stand-alone elements for controlling the polarization state of thermal radiation driven by unpolarized electromagnetic fluctuations dictated [63] by the fluctuation-dissipation theorem. On the contrary, it can be demonstrated that the 2D chiral metasurface shown in Fig. 1a transmits primarily one CP state. To see this, note that the air-side transmission through the metasurface is highly unusual as indicated by the results of the COMSOL simulations shown in Fig. 5 . For example, for a planar non-chiral interface one expects that the diagonal elements of the cross-polarized transmission matrix T α,β ( λ ) in the circularly polarized basis ( α , β : RCP or LCP) dominate over the polarization-converting off-diagonal elements for all wavelengths λ . This is clearly not the case for the studied 2D chiral metasurfaces: according to Fig. 5b the diagonal elements are very small while the off-diagonal element T LR is dominant at the resonant wavelength λ F ≈4.7 μm. Because of the resonant nature of the metasurface, the RCP-to-LCP and LCP-to-RCP transmission coefficients differ significantly at Fano resonances: T LR ≫ T RL despite that T LL ≈ T RR as expected [55] for non-3D chiral metamaterials with small substrate effects. This extreme chirality implies that, unlike in the case of a birefringent metasurface, the transmitted radiation is primarily CP even for unpolarized incident light. Depending on the position of the nanorod’s bend, the resulting CP state can be engineered to be either mostly LCP (if T LL ≈ T RR ≈0 and T LR ≫ T RL as shown in Fig. 5b ) or mostly RCP (if T LR ≪ T RL ). 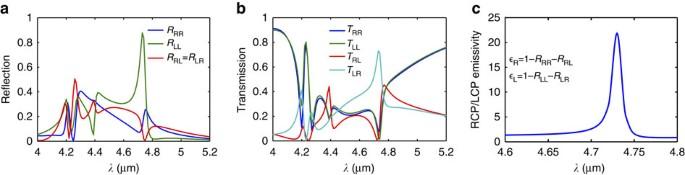Figure 5: Narrow-band thermal emission of infrared light with high DCP. (a) Numerical (COMSOL) simulation of the cross-polarized reflectivity matrixRα,βin the circularly polarized basis (α,β: RCP or LCP). Note thatRRL≡RLRby reciprocity. (b) Air-side cross-polarized transmission matrixTα,β. Note that the slight deviation fromTRR=TLLis a substrate effect in SOI-based metasurfaces:nSiO2≠nair. (c) Estimated DCP of thermal infrared radiation emitted by an infrared-absorbing slab capped by the 2D chiral metasurface. Unit cell dimensions as inFig. 1andL=1.8 μm. Figure 5: Narrow-band thermal emission of infrared light with high DCP. ( a ) Numerical (COMSOL) simulation of the cross-polarized reflectivity matrix R α,β in the circularly polarized basis ( α , β : RCP or LCP). Note that R RL ≡ R LR by reciprocity. ( b ) Air-side cross-polarized transmission matrix T α,β . Note that the slight deviation from T RR = T LL is a substrate effect in SOI-based metasurfaces: n SiO2 ≠ n air . ( c ) Estimated DCP of thermal infrared radiation emitted by an infrared-absorbing slab capped by the 2D chiral metasurface. Unit cell dimensions as in Fig. 1 and L =1.8 μm. Full size image The strong asymmetry of the total transmission of the two circular polarization states through the 2D chiral dielectric metasurface makes it very distinct from ultrathin 2D chiral metallic metasurfaces that rely on either Ohmic dissipation or symmetry-breaking substrate effects [55] , [62] to achieve such transmission asymmetry. Numerical simulations (not shown) indicate that even in the absence of substrate effects (that is, when the z→ − z special inversion symmetry is preserved) and dissipation (which is negligible in Si for mid-IR frequencies) it is possible for the total transmission of the RCP light, T R ≡ T RR + T LR , to be different from the total transmission of the LCP light, T L ≡ T LL + T RL . The physical reason for this is that the combination of spatial inversion and time reversal symmetries only enforces the T LL ≡ T RR requirement. The T LR ≠ T RL inequality does not violate any symmetry and does indeed occur for all-dielectric metasurfaces with small but finite thickness. In fact, it can be shown that a lossless all-dielectric metasurface shown in Fig. 1 embedded in a fully symmetric dielectric environment can be designed to satisfy the following transmission property at a specific wavelength: T LL = T RR = T RL =0 and T LR ≠0. Satisfying these conditions of extreme chirality ensures that T L =0 while T R ≠0, making the metasurface a functional equivalent of an optical device comprising a quarter-wave plate with principal optical axes ( x ′, y ′), followed by a linear polarizer whose transmission axis is titled at 45° with respect to ( x ′, y ′), followed by an identical quarter-wave plate. Remarkably, this functionality is achieved by a metasurface that is only about a micron thick. Such functionality cannot be accomplished by an ultrathin 2D chiral metallic metasurface because the continuity of the electric field across the metasurface enforces the T LR = T RL condition for lossless metallic metasurfaces [55] , [62] embedded in a symmetric dielectric environment. Even more significant are the implications of strong spectrally selective reflection asymmetry ( R LL ≠ R RR as shown in Fig. 5a ) for applications involving thermal emission of circularly polarized states of light because the emissivity is related to the surface reflectivity through Kirhhoff’s law. For example, the circularly polarized emissivity coefficients ε R ( λ ) and ε L ( λ ) for a bulk-absorbing emitter can be expressed as ε R =1− R RR − R LR and ε L =1− R LL − R RL . Thus, calculated CP emissivity coefficients plotted in Fig. 5c show a high DCP( λ )≡ ε R / ε L of the thermal emission at the Fano resonance wavelength λ F : DCP( λ ) has a spectral FWHM of δλ FWHM ≈30 nm and the peak value of DCP( λ F ) >20, which is almost two orders of magnitude higher than its baseline value outside of this narrow resonance region. Additional examples of metasurfaces designed to perform as spectrally selective thermal emitters of CP IR radiation are shown in Supplementary Fig. 2 . The unique spectral (very narrow band) and polarization (high DCP) characteristics of the thermal radiation produced by the proposed 2D chiral metasurfaces suggest their applications to IRID tag technologies because they can be easily distinguished from the unpolarized thermal radiation emitted by the environment, and because multiple narrow emission bands with high DCP can be used within the atmospheric transparency window (3 μm< λ <5 μm). Although fully-3D helical metamaterials [8] or their multilayer equivalents [9] can potentially deliver similar performance, their fabrication is considerably more complex than that of a single-layer micron-thick metasurface described here. High-quality factor and large optical concentration suggest that the above considered metasurfaces could be employed as an excellent platform for enhancing light–matter interaction and for sensing/spectroscopy of minute quantities of matter. 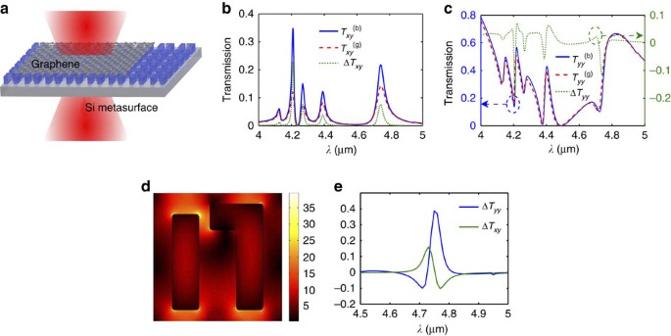Figure 6: Atomic/molecular monolayer sensing using Si metasurfaces. (a) A schematic of detecting a single layer of graphene using the silicon metasurface. (b) Cross-polarized transmissionTxybefore () and after () metasurface functionalization with single-layer graphene with the Fermi level ofEF=0 eV.is the transmission reduction because of graphene. (c) Same as (b), but fory-polarized transmissionTyyand graphene’s Fermi level ofEF=0.3 eV. (d) The calculated near-field enhancement, |E|/|Ein|, corresponding to the TM100resonance. The field amplitude is plotted along thez=600 nm plane, wherez=0 nm is the Si/SiO2interface. (e) Calculated difference spectra induced by a 10-nm protein layer covering the silicon metasurface. The protein layer is assumed to have an optical refractive indexn=1.5. Unit cell dimensions: as inFig. 1andL=1.8 μm. Figure 6d shows the calculated near-field enhancement around the silicon metasurface at the Fano resonance wavelength λ F ≈4.7 μm corresponding to the TM 100 mode (unit cell parameters: same as in Fig. 5 ; field distributions for other dark modes are shown in Supplementary Note 2 ). Large optical intensity enhancement comparable to that obtained in plasmonic Fano-resonant metasurfaces [12] and distributed over a considerable fraction of the nanorods’ surface, combined with high spectral selectivity of the all-dielectric metasurface suggests that even minute matter quantities placed at or near the nanorods’ surface can strongly affect the transmission. Figure 6: Atomic/molecular monolayer sensing using Si metasurfaces. ( a ) A schematic of detecting a single layer of graphene using the silicon metasurface. ( b ) Cross-polarized transmission T xy before ( ) and after ( ) metasurface functionalization with single-layer graphene with the Fermi level of E F =0 eV. is the transmission reduction because of graphene. ( c ) Same as ( b ), but for y -polarized transmission T yy and graphene’s Fermi level of E F =0.3 eV. ( d ) The calculated near-field enhancement, | E |/| E in |, corresponding to the TM 100 resonance. The field amplitude is plotted along the z =600 nm plane, where z =0 nm is the Si/SiO 2 interface. ( e ) Calculated difference spectra induced by a 10-nm protein layer covering the silicon metasurface. The protein layer is assumed to have an optical refractive index n =1.5. Unit cell dimensions: as in Fig. 1 and L =1.8 μm. Full size image As one representative example, we consider the enhancement of the interaction of infrared light with SLG without the need to focus infrared light to wavelength-scale spots [21] . The optical response of metal-based antennas [64] , [65] and metasurfaces [57] has been modified by combining them with SLG, and the extracted information was further used to estimate the carrier density in SLG [57] . However, as the spectral linewidth of metal-based structures is fairly broad, only modest changes of the optical response (transmission or reflection) of metasurfaces have been accomplished so far. Our numerical simulations demonstrate that much stronger SLG-induced modification of the transmission through the high- Q non-metallic metasurfaces can be obtained. To demonstrate the effect of SLGs with different free-carrier densities (parameterized by the corresponding values of the Fermi energy E F ) placed on top of a metasurface as shown in Fig. 6a , we numerically investigated the induced transmission changes in T xy and T yy . The two limiting cases shown in Fig. 4b,c correspond to E F =0 (interband transitions in SLG make its conductivity real [66] and cause light absorption) and E F =0.3 eV (interband transitions are Pauli-blocked; however, intra-band transitions cause graphene’s inductive response and the blue-shifting of Fano resonances). Significant changes in T xy and T yy near Fano resonances found in both limiting cases demonstrate that silicon metasurfaces can be used as a novel platform for spectroscopic characterization of SLG. As the second representative example, we consider the effect of conformally coating protein monolayers on the optical response of Si-based metasurfaces. Those can be readily functionalized by proteins and protein monolayers that naturally attach to the native oxide formed on the metasurface. An example of the modified transmission spectra (with and without a 10-nm protein on the metasurface) is shown in Fig. 6d . Note a remarkable Δ T yy ≈40% transmission change, indicating that submonolayer quantities of protein matter can be detected using Fano-resonant dielectric metasurfaces. The high- Q Fano-resonant dielectric metasurfaces described here represent a novel and promising platform for a variety of applications that depend on high optical energy enhancement and precise spectral matching between molecular/atomic and electromagnetic resonances. Those include infrared spectroscopy of biological and chemical substances and nonlinear infrared optics. Chiral properties of such metasurfaces might be exploited for developing novel ultrathin infrared detectors sensitive to light’s chirality, as well as spectrally selective CP thermal emitters [61] . Even higher quality factors ( Q >1,000) Fano-resonant metasurfaces can be developed by judicious engineering of near-field coupling between resonant modes if inhomogeneous broadening because of fabrication imperfections can be overcome. Combining the large-field enhancements achieved in such high- Q silicon metasurfaces with coherent radiation sources such as quantum cascade lasers capable of delivering high-power low-divergence beams [67] would open new exciting opportunities in nonlinear infrared optics such as harmonics generation and four-wave mixing [13] , [14] using free-space excitation. Sample preparation The samples were fabricated by performing inductively coupled plasma etching on double-layered SOI wafers, with the thickness of each layer being h 1 =1.2 μm (Si), h 2 =1.6 μm (SiO 2 ), h 3 =1.2 μm (Si) and h 4 =1.6 μm (SiO 2 ). Only the top active silicon layer is etched into the designed nanorod arrays. The double-layered SOI substrates were patterned in a JEOL JBX-6300FS electron beam lithography system using the NEB-31A-negative resist. After post baking and development, inductively coupled plasma etching was used to obtain the final nanostructures. The nanostructures were etched using an Ar/HBr plasma chemistry as it has high Si to SiO 2 selectivity, after a brief Ar/Cl 2 oxide break through-etch. The sample etch was monitored via an end point detection laser and it ended with an additional 25% over etch to ensure that Si was removed sufficiently in the patterned regions. The schematic and dimensions of the SOI wafer are shown in Supplementary Fig. 3 . Optical measurements All cross-polarized optical spectra were acquired using a Thermo Scientific Nicolet 6700 FTIR spectrometer. The collimated IR beam emerging from the FTIR spectrometer is passed through the image-forming pinhole, a wire-grid polarizer, focused normally on the metasurface using an aspherical ZnSe lens, and then on an MCT detector placed behind an analyser. Stokes parameters of the silicon metamaterials The polarization state of the transmitted y -polarized incident light was experimentally investigated using the standard rotating analyser Stokes polarimetry setup [59] illustrated in Fig. 4a . The transmission spectra were acquired by varying the analyser orientation with a 10° step from φ =0° to φ =90°. If the polarization state of the transmitted light is given by , then the time-averaged intensity the analyser is given by . The three parameters, E 0 , θ E and the absolute value of φ E can therefore be determined by fitting the measured intensity as a function of φ , and then used to express the polarization state of light in terms of the more familiar Stokes parameters: , and . The nonzero S 3 corresponds to elliptically polarized light, and S 3 =± S 0 corresponds to right/left circularly polarized light. The measured and theoretically calculated Stokes parameters for all three metasurfaces with L =1.6, L =1.8 and L =2.0 μm are shown in Supplementary Fig. 1 . The initially polarized light is, in general, elliptically polarized after the passage through the metasurface. The principal dimensions of the polarization ellipse, its tilt angle β and the ratio a / b between its long and short axes defined in Fig. 4b can be expressed in terms of the Stokes parameters as follows. The tilt angle of the ellipse, β , is calculated according to tan2 β =tan2 θ E cos φ E = S 2 / S 1 , and the ellipticity is given by . The inverse ellipticity, b / a , and the tilt angle of the transmission are plotted in Supplementary Fig. 4 for all three metasurfaces. In all experiments the incident field is kept linearly polarized along the y direction. Numerical simulations We used the finite element solver, COMSOL, to simulate the electromagnetic response of the fabricated structures. The simulation domain includes one unit cell of the structure with periodic boundary conditions in both x and y directions. Perfectly matched layers are set in the z direction with a current sheet to generate the incident field. The permittivity of Si and SiO 2 are taken from ref. 68 . Estimation of the quality factors from the measured spectra Table 1 lists the estimated quality factors of the metasurface resonances. The quality factors, , are estimated by fitting the measured T xy spectra with a Lorentzian lineshape given by . In typical Fano resonances, the Q-factors should be obtained through fitting with the Fano lineshape given by , where a 1 is in general a complex number. In our case, the Fano resonance involves polarization conversion because of the strong chirality. The consequence is that the y -polarized incident light will be partially converted into x -polarized transmission at the Fano resonances. As can be seen in Fig. 3 of the manuscript, T xy exhibits near-Lorentzian peaks at the Fano resonances, while T yy exhibits typical non-symmetric Fano lineshape. We therefore chose to fit T xy with Lorentzian curves to reduce the number of fitting parameters. Strictly speaking, the T xy spectra are still Fano lineshapes but with very small background, a 1 →0. In Supplementary Fig. 5 , we compared both the Lorentzian and the Fano fittings to the measured T xy for the TM 100 mode. It is shown that the two fittings are giving consistent estimation for the Q- factors. In Supplementary Fig. 6 , we fitted the measured extinction spectra (1− T xx and 1− T yy ) using a Fano model: , in which x 2 and x 3 are the resonant frequency and the damping rate for the bright mode, respectively, and x 6 and x 7 are the corresponding quantities for the dark mode. The following results were obtained for the x -polarized extinction: The wavelength of the bright mode for the x -polarized extinction μm, and the Q- factor for the x -polarized extinction given by Q = x 6 / x 7 /2 is found to be Q xx ≈98.6. The corresponding fitting data for the y -polarized extinction is given by The wavelength of the bright mode for the y -polarized extinction μm, and the Q factor for the y- polarized extinction given by Q = x 6 / x 7 /2 is found to be Q xx ≈85.2. These values of the Q -factor are close to the Q -factor of 94.3 estimated using the almost-Lorentzian cross-polarized transmission spectra. The spectral position of the dark resonance is essentially identical for all three extraction methods. 2D chirality We calculated the transmission of circular polarized light through the silicon metamaterials. The results are shown in Supplementary Fig. 7 for the three samples with L =1.6, 1.8 and 2 μm. The incident fields are either RCP or LCP, with a 90° incident angle. The transmission coefficients are denoted by T ij , with i , j =R or L being the polarization of the transmitted and the incident light, respectively. It is shown that T RL ≠ T LR near the dark resonances, indicating 2D chirality of the structures. Likewise, reflectivities from a 2D chiral surface can also be highly asymmetric. For example, the polarization-converting reflectivities R RR ( λ ) (from incident RCP to reflected RCP) can be substantially different from R LL ( λ ) (from incident LCP to reflected LCP) in 2D chiral metasurfaces. On the other hand, the non-chiral reflectivities are equal ( R RL ( λ )= R LR ( λ )). Both chiral and non-chiral reflectivities are plotted in Supplementary Fig. 2 . The non-equal chiral reflectivities have important implications for circularly polarized infrared emissivity from 2D metasurfaces. Such asymmetry can produce considerable asymmetry between emissivities of RCP and LCP light close to Fano resonances as shown in Supplementary Fig. 2 . Note that the mirror-like (non-chiral) reflectivity is very low for both left- and right-hand circular polarizations. Our calculation of circularly polarized emissivities indicates high DCP thermally emitted by the meta-surface. The calculation assumes that all radiation transmitted through the meta-surface is eventually absorbed inside the substrate. Note that outside of the very narrow Fano resonance band ( δλ FWHM ≈25 nm) thermal radiation is not circularly polarized. Comparison between metal and silicon-based metasurfaces Low loss in crystalline silicon is the key enabler of the ultrahigh quality resonances described in this manuscript. To make a meaningful comparison, we have fabricated plasmonic metasurfaces with similar topology to the silicon-based structures shown in Fig. 1 . The results of the comparison are shown in Supplementary Fig. 8 , where the cross-polarized transmission T xy ( λ ) is plotted for two different plasmonic metasurfaces and two silicon-based metasurfaces. The two plasmonic metasurfaces differ by their Q- factors that are controlled by the positioning of the horizontal stub along the length of the right antenna. Even leaving the amplitude of the T xy ( λ ) aside, it is obvious from Supplementary Fig. 8 that the Q -factors of the silicon-based metasurfaces are about an order of magnitude higher than those of the plasmonic ones because of lower non-radiative losses in the former. Spectra acquired using an infrared microscope and a collimated beam Quality factors of coherent Fano resonances are sensitive to the divergence angle Δ θ of the incident light, as well as to the absolute value of the incidence angle θ . Those are determined by the focusing optics, as well as by the angular size of the thermal radiating source in the case of the infrared beams that are not diffraction-limited. Maintaining small values of Δ θ and θ is essential for maintaining low radiative losses of the dark modes. Those are determined by the intrinsic asymmetry of the unit cell (governed by the length L x = d − g ≈500 nm of the antenna’s bend) and the phase retardation φ x =2 πd sin( θ )/ λ between the antennas (governed by the incidence angle θ ). The condition of low radiative losses places considerable constraints on the beam’s quality and, more importantly, on the focusing optics used to focus the beam on the sample. The effect of the focusing optics on the excitation of ultrasharp Fano resonances is best illustrated by comparing the cross-polarized transmission spectra T xy ( λ ) acquired using an infrared microscope (corresponding to high-NA focusing optics) and using a collimated infrared beam with small angular divergence focused by low-NA ZnSe lens. Both beams are coupled to the same FTIR spectrometer, but the latter is coupled to FTIR’s external port and focused using external focusing optics as illustrated in the inset to Supplementary Fig. 9 . The details of the external setup are described elsewhere [69] . As shown in Supplementary Fig. 9 , the spectral features of T xy ( λ ) acquired using a collimated beam with the measured divergence angle Δ θ ≈7° are considerably sharper and stronger than those acquired using a microscope because the latter has a considerable angular divergence and large incidence angle produced by high-NA Cassagraine focusing optics of the microscope. How to cite this article: Wu, C. et al. Spectrally selective chiral silicon metasurfaces based on infrared Fano resonances. Nat. Commun. 5:3892 doi: 10.1038/ncomms4892 (2014).